Controlled thermal oxidative crosslinking of polymers of intrinsic microporosity towards tunable molecular sieve membranes Organic open frameworks with well-defined micropore (pore dimensions below 2 nm) structure are attractive next-generation materials for gas sorption, storage, catalysis and molecular level separations. Polymers of intrinsic microporosity (PIMs) represent a paradigm shift in conceptualizing molecular sieves from conventional ordered frameworks to disordered frameworks with heterogeneous distributions of microporosity. PIMs contain interconnected regions of micropores with high gas permeability but with a level of heterogeneity that compromises their molecular selectivity. Here we report controllable thermal oxidative crosslinking of PIMs by heat treatment in the presence of trace amounts of oxygen. The resulting covalently crosslinked networks are thermally and chemically stable, mechanically flexible and have remarkable selectivity at permeability that is three orders of magnitude higher than commercial polymeric membranes. This study demonstrates that controlled thermochemical reactions can delicately tune the topological structure of channels and pores within microporous polymers and their molecular sieving properties. Microporous materials with well-defined size-selective channels and pores are promising next-generation molecular sieving materials for gas sorption, storage and separations [1] , [2] , [3] . Inorganic and organic ordered open frameworks, such as zeolites [4] , [5] , [6] , [7] , and metal–organic frameworks (MOFs) [8] , [9] , [10] , are representative microporous molecular sieving materials with precisely defined pore architecture. Owing to their tailored pore size, chemical functionality and high surface area, these ordered frameworks are promising for gas sorption [8] , [9] , [10] , storage [11] , catalysis [12] , adsorption-based separations [13] and potentially have excellent intrinsic selectivity and permeability in membrane separations [6] , [7] . However, these crystalline frameworks are generally brittle and suffer from difficulty in manufacturing to large scale separation membranes [14] . In contrast, industrial selective membranes are made of solution-processable densely packed polymers where molecular transport follows a solution diffusion mechanism, and presents a trade-off between permeability and selectivity [15] , known as an upper bound [16] , [17] , as shown in an overview figure ( Fig. 1g ). Solution-processable and microporous molecular sieving materials are desirable for the next-generation high-performance membranes to achieve both high permeability and high selectivity. 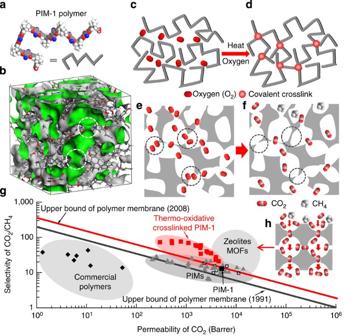Figure 1: Polymer molecular sieves. (a) An ideal molecular model of a polymer of intrinsic microporosity (PIM-1) polymer chain segment. (b) Three-dimensional view of an amorphous cell of PIM-1 polymer (four polymer segments inside, each containing 10 repeating units). Cell size: 31.8 × 31.8 × 31.8 Å, apparent bulk density of 1.050 g cm−3. The grey surface indicates the van der Waals surface, green surface is the Connolly surface with probe radius of 1.65 Å. Dashed circles indicate the bottlenecks between interconnected cavities. (c,d) Two-dimensional schematic illustration of thermal oxidative crosslinking of (c) independent rigid polymer chains (black contorted lines) to (d) covalently crosslinked polymer network via thermal treatment at suitable temperatures (350–450 °C) in the presence of trace amount of oxygen molecules. (e) Two-dimensional schematic illustration of pore topologies in microporous polymer membranes and (f) thermal-oxidatively crosslinked polymer membranes with narrower or closed gate (indicated by dashed circles) between interconnected cavities, which give better size and shape selectivity (for example, separation of CO2from CH4). White regions indicate the accessible free volume, grey regions indicates the inaccessible pore walls (occupied by polymer chains). (g) The upper bound plot of selectivity versus permeability for conventional dense polymeric membranes, and microporous molecular sieving membranes, as represented by amorphous PIMs and ordered molecular sieves (MOFs and zeolites) illustrated in inset ofh. The upper bounds were summarized by Robeson in 1991 (ref.16) and 2008 (ref.17), respectively. Figure 1: Polymer molecular sieves. ( a ) An ideal molecular model of a polymer of intrinsic microporosity (PIM-1) polymer chain segment. ( b ) Three-dimensional view of an amorphous cell of PIM-1 polymer (four polymer segments inside, each containing 10 repeating units). Cell size: 31.8 × 31.8 × 31.8 Å, apparent bulk density of 1.050 g cm −3 . The grey surface indicates the van der Waals surface, green surface is the Connolly surface with probe radius of 1.65 Å. Dashed circles indicate the bottlenecks between interconnected cavities. ( c , d ) Two-dimensional schematic illustration of thermal oxidative crosslinking of ( c ) independent rigid polymer chains (black contorted lines) to ( d ) covalently crosslinked polymer network via thermal treatment at suitable temperatures (350–450 °C) in the presence of trace amount of oxygen molecules. ( e ) Two-dimensional schematic illustration of pore topologies in microporous polymer membranes and ( f ) thermal-oxidatively crosslinked polymer membranes with narrower or closed gate (indicated by dashed circles) between interconnected cavities, which give better size and shape selectivity (for example, separation of CO 2 from CH 4 ). White regions indicate the accessible free volume, grey regions indicates the inaccessible pore walls (occupied by polymer chains). ( g ) The upper bound plot of selectivity versus permeability for conventional dense polymeric membranes, and microporous molecular sieving membranes, as represented by amorphous PIMs and ordered molecular sieves (MOFs and zeolites) illustrated in inset of h . The upper bounds were summarized by Robeson in 1991 (ref. 16 ) and 2008 (ref. 17 ), respectively. Full size image Microporous polymers are a relatively new class of materials that are attractive for applications as organic molecular sieves [18] , [19] , [20] , [21] . Polymers of intrinsic microporosity (PIMs) [20] , [21] , [22] , [23] , [24] , [25] , [26] , [27] , invented by Budd and McKeown and coworkers, are a novel subclass of microporous polymers with unique rigid and contorted macromolecular backbone structure (for example, PIM-1 in Fig. 1a , chemical structure is given in the Supplementary Fig. 1 ). The poor molecular packing of such rigid chains results in disordered heterogeneous material with regions of irregularly shaped free volume at molecular dimensions in the solid state, as visualized by the molecular simulation ( Fig. 1b ). The fractional free volume in PIMs is sufficiently high that free volume elements are effectively interconnected, behaving like micropores (pore dimensions below 2 nm) according to the definition of IUPAC. Such high free volume allows the high solubility of gas molecules, while the bottleneck or gates interconnecting micropores behave as sieves for gas molecules with different size and shape. Such interconnected microporosity is analogous to the pore structure of ordered molecular sieves (for example, zeolites), as schematically illustrated in Fig. 1h . The structure of the interconnected cavities in PIMs materials are also thought to resemble the hour-glass shaped channel systems in naturally occurring biological membranes, such as water channels (known as Aquaporin) [28] , and ion channels [29] . Cell membranes utilize such unique channels for rapid molecular and ion transport while providing a chemically gated selection mechanism. Similarly, the unique micropore structure of PIMs materials offers remarkable combinations of permeability and selectivity that surpass the upper bound of synthetic polymer membranes. In contrast to crystalline molecular sieves, microporous polymers are generally amorphous and flexible. Linear polymer chains interacting by relatively weak van der Waals forces or entanglements could easily slide over each other. In addition, molecular modelling of PIM-1 indicates that the spirobisindane unit and dioxane linkages are relatively flexible [30] . This amorphous and flexible nature of PIMs polymer chains results in a broad size distribution of free volume elements (for example, 4–10 Å), which compromises their separation performance, for example, poor molecular selectivity, physical aging and plasticization. As indicated by theoretical prediction by Freeman [15] , there are two strategies to enhance both the permeability and selectivity of polymeric membrane materials. One approach is improving the solubility selectivity ( S A / S B ), such as PIMs substituted with CO 2 -philic tetrazole groups (TZ–PIMs) [20] . An alternative approach is increasing the rigidity of polymer chains while maintaining large interchain spacing, such as thermal rearranged (TR) polymers [18] , [31] , and PIMs with more rigid backbone [21] , [32] , [33] , [34] , for example, PIMs containing rigid Troger’s Base (TB) units [21] , and triptycene-based PIMs [33] , [34] . In particular, for separations of industrially and environmentally important gases, such as condensable CO 2 and hydrocarbons in natural gas, all of the existing PIMs polymers have only shown modest selectivity (for example, selectivity of CO 2 /CH 4 ~10). Therefore, tailoring the distribution, size and architecture of channels and pores is critical to achieve a substantial increase of selectivity. A typical feature of polymers, as soft materials, is their deformability under external stimulus (for example, light, heat, oxidant and stress, and so on), and even very mild deformation would induce significant change of physical properties. Recently, we reported the photooxidative degradation of PIM-1 polymer on exposure to ultraviolet light irradiation in the presence of oxygen, which induces oxidative chain scission and local densification at the surface [35] . Similarly, thermo-oxidative degradation or crosslinking could occur for PIM-1 polymer when polymers are heated in the presence of oxygen. The oxidative degradations of conventional polymers are well known, but very limited studies on PIMs polymer materials have been reported. An earlier paper by Li et al. [36] of the Chung group described thermal processing of PIM-1 at 300 °C over a period of 1–2 days and reported the simultaneous increase of both permeability and selectivity. The work by Li et al. was described as being done within a vacuum oven with no information on the environment in terms of pressure or O 2 concentration. However, PIM-1 was reported to be thermally stable at temperatures up to 450 °C in inert atmosphere (350 °C in air), according to the initial work by Budd et al. [23] . In this work, using PIM-1 as a prototypical microporous polymer, we demonstrate a simple process of thermal oxidative crosslinking of independent rigid polymer chains to covalently crosslinked polymer networks with significantly enhanced molecular-sieving selectivity and exceptional gas separation performance. From a microscopic point of view, as schematically shown in Fig. 1c–f , the high free volume polymer matrix behaves as a series of interconnected nano reactors, which allows sorption and fast diffusion of oxygen molecules through the gates between the interconnected cavities. On heating in a suitable temperature window (350–450 °C) in the presence of trace amounts of oxygen, we hypothesize that oxidative crosslinking of polymer chains occurs at the larger bottlenecks of interconnected micropores owing to the preferential diffusion of oxygen. Such a vulcanization process results in three-dimensional crosslinked networks with narrower (or closed) gates offering remarkably better size and shape selectivity while the overall free volume is still sufficiently high, allowing rapid and selective diffusion of gas molecules. Characterization of membranes We fabricated free-standing dense PIM-1 membranes (thickness ~50 μm) by casting the solution of polymer ( Fig. 2a ). After thermal oxidative crosslinking at 385 °C in the presence of trace amounts of oxygen (vacuum of 1 mbar) for prolonged periods (up to 24 h), the transparent membrane changed from fluorescent yellow ( Fig. 2b ) to dark brown as visually observed ( Fig. 2c ). The thermal-oxidatively crosslinked PIM-1 (termed as TOX-PIM-1 hereafter) polymer membranes became largely insoluble (gel content >95%) in solvents that readily dissolve the PIM-1 polymer, such as chloroform ( Fig. 2d ), tetrahydrofuran or dichloromethane (details of solubility tests are given in Supplementary Fig. 2 ). Furthermore, ultraviolet–visible absorption spectra and loss of photoluminescence of polymer films clearly indicate the degradation of polymer ( Supplementary Fig. 3 ). The membranes showed weight loss of ~2 wt% owing to the thermal oxidative degradation. The skeletal density of crosslinked membranes slightly increased from 1.335±0.006 to 1.365±0.007 g cm −3 , while there is no substantial change in apparent bulk density (1.060–1.100 g cm −3 ). Wide-angle X-ray scattering confirms TOX-PIM-1 polymers remain amorphous ( Supplementary Fig. 4 ). Thermogravimetric analysis indicated high thermal stability of both PIM-1 and TOX-PIM-1 up to ~450 °C in an inert argon atmosphere ( Supplementary Fig. 5 ). As examined by scanning electron microscopy (SEM) ( Supplementary Fig. 6 ), both PIM-1 and TOX-PIM-1 polymer membranes are defect free and do not show observable mesoporosity; therefore, the gas transport properties as measured are intrinsic values. 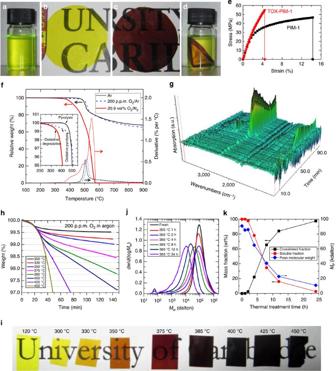Figure 2: Characterization of polymer membranes. (a) Photo of PIM-1 polymer solution in chloroform. (b) Photo of as-prepared PIM-1 membrane. (c) Photo of thermal-oxidatively crosslinked (TOX) PIM-1 membrane and (d) solubility test in chloroform. (e) Stress–strain curve of PIM-1 and TOX-PIM-1 membranes. (f) Thermogravimetric analysis of PIM-1 polymer membranes in argon (black), 200 p.p.m. O2in argon (blue) and air (red). Samples were heated to 1,000 °C at 10 °C min−1, and (g) correspondingin situFTIR spectra of gaseous products in argon atmosphere. (h) Weight loss profiles of isothermal oxidative degradation of PIM-1 membranes in 200 p.p.m. O2/argon, in the temperature range of 300–450 °C (full profiles are shown inSupplementary Fig. 10). (i) Photos of polymer films after isothermal oxidative crosslinking in 200 p.p.m. O2/argon for 2 h at temperatures corresponding toh. (j) Molecular weight distribution of soluble fraction of TOX-PIM-1 polymer membranes. (k) Gel content analysis and peak molecular weight of soluble fraction. The polymer membranes were heated at 385 °C under continuous vacuum (1 mbar) up to 24 h. Figure 2: Characterization of polymer membranes. ( a ) Photo of PIM-1 polymer solution in chloroform. ( b ) Photo of as-prepared PIM-1 membrane. ( c ) Photo of thermal-oxidatively crosslinked (TOX) PIM-1 membrane and ( d ) solubility test in chloroform. ( e ) Stress–strain curve of PIM-1 and TOX-PIM-1 membranes. ( f ) Thermogravimetric analysis of PIM-1 polymer membranes in argon (black), 200 p.p.m. O 2 in argon (blue) and air (red). Samples were heated to 1,000 °C at 10 °C min −1 , and ( g ) corresponding in situ FTIR spectra of gaseous products in argon atmosphere. ( h ) Weight loss profiles of isothermal oxidative degradation of PIM-1 membranes in 200 p.p.m. O 2 /argon, in the temperature range of 300–450 °C (full profiles are shown in Supplementary Fig. 10 ). ( i ) Photos of polymer films after isothermal oxidative crosslinking in 200 p.p.m. O 2 /argon for 2 h at temperatures corresponding to h . ( j ) Molecular weight distribution of soluble fraction of TOX-PIM-1 polymer membranes. ( k ) Gel content analysis and peak molecular weight of soluble fraction. The polymer membranes were heated at 385 °C under continuous vacuum (1 mbar) up to 24 h. Full size image Mechanical properties We found that thermal-oxidative treatment at a temperature of 375–385 °C along with slow thermal oxidation rate at p.p.m.-level concentrations of oxygen for a prolonged exposure time resulted in almost fully covalently crosslinked films that remained transparent, flexible and mechanically resilient. A typical plot of stress–strain curve ( Fig. 2e ) shows that the TOX-PIM-1 polymer films after slow crosslinking become stiff but are still mechanically robust in terms of tensile strength (50–60 MPa), elongation strain at break (in the range of 4–8%), and Young’s modulus (1.2 to 1.7 Gpa) ( Supplementary Fig. 7 and Supplementary Table 1 ). Nanoindentation confirmed the increase of hardness from 149±4.0 to 188±3.0 MPa while the Young’s modulus only shows a slight increase from 1.876±0.029 to 1.885±0.039 GPa ( Supplementary Fig. 8 ). For PIM-1 films annealed at higher concentrations of oxygen (for example, 20.9 vol.% O 2 in air), the films became brittle because of excessive oxidation. For the films annealed at higher temperatures (>400 °C) for prolonged periods, the samples became too brittle for stretching measurement as excessive crosslinking or degradation had occurred. Thermal oxidative crosslinking We confirmed the critical role of oxygen in thermal-oxidative degradation and crosslinking of the polymer membranes. PIM-1 polymer is thermally stable in inert atmosphere, with evident degradation at temperatures above 450 °C in pure argon ( Fig. 2f ). In situ Fourier transform infrared (FTIR) spectra of gaseous products evolved during pyrolysis in thermogravimetric analyser (TGA) ( Fig. 2g ) indicates that the scission of ether linkages in the backbone is the dominant decomposition step since only dioxane linkages are the oxygen-containing groups, generating CO 2 as primary gaseous product (2,260 cm −1 in the spectra), although the initiation step is not clear. In contrast, thermal-oxidative degradation of the PIM-1 polymer occurs at much lower temperature, with evident oxidation starting at 350 °C in air ( Fig. 2f ) and CO 2 as major gaseous product ( Supplementary Fig. 9 ). Such oxidative degradation was confirmed by baking the polymer membranes in an oven at the same temperature in air. Alternatively, exposing the membranes in air in the temperature range of 300–450 °C for prolonged periods could result in varied degree of oxidative degradation (for example, complete degradation with CO 2 as primary product, Supplementary Fig. 9 ). Therefore, there is a temperature window between 350–450 °C where oxidative pyrolysis could occur, as confirmed by heating PIM-1 polymer in inert purging gas at low O 2 concentrations (for example, 200 p.p.m. O 2 ) ( Fig. 2f ). These experiments confirm the dominant mechanism of thermal-oxidative degradation in the presence of oxygen. We further tuned the degree of thermal-oxidative crosslinking of PIM-1 polymer using a reaction engineering approach, via changing the O 2 concentration, temperature and reaction time, and tracked the evolution of gel content and molecular weight distribution. For example, the polymer heated in argon containing 200 p.p.m. O 2 at 300–450 °C underwent oxidative crosslinking and pyrolysis ( Fig. 2h and Supplementary Fig. 10 ), rather than significant degradation in air. As the reaction temperature increase, the films changed from fluorescent yellow to dark brown and black ( Fig. 2i ). Characterization of these samples indicate similar physical and chemical properties as those obtained in a vacuum oven for prolonged time, although they are relatively more brittle due to the high O 2 concentration (200 p.p.m.). These TGA experiments confirmed that the optimal crosslinking temperature appears to be around 375–385 °C (tunable depending on the O 2 concentration), and a weight loss of 1.5–2.5 wt% due to thermal oxidation would be sufficient to induce crosslinking. Therefore, we are able to tune the extent of oxidation and crosslinking based on Arrhenius-like chemical reaction kinetics ( Supplementary Note 1 and Supplementary Fig. 11 ), and terminate the reaction at the suitable point under controlled conditions, to avoid excessive degradation or carbonization. The thermal-oxidatively crosslinked polymer films were dissolved in chloroform, as shown in Fig. 2d , with non-dissolved gel and soluble solution separated. The molecular weight distribution in the soluble polymer solution, evolves from a peak molecular weight of 100 kDa to a disperse mixture of fragments of molecular weight up to several hundred ( Fig. 2j ), indicating that random oxidative chain scission occurred involving the backbone. At the same time, the weight fraction of insoluble gel content increased ( Fig. 2k ); therefore, we propose that oxidative chain scission and in situ covalent crosslinking occurred. Similar changes were observed for the polymer films exposed to varied temperatures ( Supplementary Fig. 12 ). Furthermore, ex situ FTIR spectra ( Supplementary Fig. 13 ) of TOX-PIM-1 polymer films confirmed that the membranes remain in the polymeric state rather than being carbonized, but the presence of weak peaks corresponding to residual carbonyl and weak hydroxyl groups provides a clear evidence of oxidation. The nitrile (C≡N) groups are relatively stable and peaks associated with C=N groups were not observable, an evidence denying the mechanism of trimerization. To summarize, these characterization analyses suggest a thermal-oxidative degradation mechanism following reaction pathways of free radicals induced oxidative chain scission, and in situ covalent crosslinking. In addition to covalent crosslinking bonds, the local oxidation of polymer may also introduce intermolecular or intramolecular interactions via hydrogen bonding between ether linkages of the backbone and residual oxidized groups (for example, carboxylic acid) in polymer chains ( Supplementary Fig. 14 ), as experimentally observed in carboxylated PIMs [37] . The hydrogen bonding could form physical crosslinking and tighten the chains locally in the polymer matrix, along with the covalent crosslinking bonds. Gas sorption properties The gas solubility in polymer membranes was probed with a series of gas sorption measurements. Low temperature gas sorption/desorption is a widely used method to probe the pore structure of microporous materials; however, it is not very effective for microporous polymers. In particular, the N 2 adsorption of TOX-PIM-1 membranes at 77 K shows an unexpected gate-opening effect, as shown in Fig. 3a , which is related to the kinetically limited diffusion of N 2 molecules through the dynamically open-and-shut gates connecting free volume elements, as illustrated in Fig. 1e . Such a gate-opening phenomenon indicates the complicated molecular interactions at low temperature (77 K), and although it has been reported in other works, it is not well understood for PIM-1 and other high free volume polymers [38] , [39] . Gas sorption properties of CO 2 , CH 4 and N 2 were also measured at 273 K ( Fig. 3b ). The TOX-PIM-1 polymer membrane showed slightly lower CO 2 sorption than that of PIM-1. Pore size distributions derived from CO 2 sorption isotherms at 273 K based on non-local density functional theory methods ( Supplementary Fig. 15 ) show an apparent loss of ultra microporosity (size smaller than 7 Å), in agreement with our proposed mechanism of narrower bottlenecks of the interconnected micropores. At room temperature (295 K), gas sorption isotherms ( Fig. 3c ) follow the dual mode sorption mechanism without observable plasticization at high pressure. The solubility of various gases (295 K, 1 bar) in TOX-PIM-1 was not significantly altered from the unmodified PIM-1. 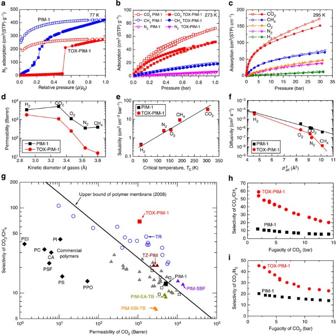Figure 3: Gas sorption and transport properties. (a) N2adsorption–desorption isotherms at 77 K. (b) Gas sorption isotherms at 273 K and (c) high-pressure gas sorption at 295 K (open symbols: PIM-1 membrane; solid symbols: TOX-PIM-1 membrane). (d) Permeability versus kinetic diameter of gases measured at 295 K. (e) Gas solubility (1 bar, 295 K) as a function of critical temperature (TC) of gas molecules. (f) Diffusivity as a function of square of effective molecular diameter (deff) of gas molecules at 295 K. (g) Robeson plot of CO2/CH4selectivity versus CO2permeability. Commercial polymers are included for comparison: cellulose acetate (CA); ethyl cellulose (EC); polycarbonate (PC); Matrimid 5218 polyimide (PI); polyetherimide (PEI); polyphenyleneoxide (PPO); polysulphone (PSF), for comparison see ref.40. Upper bound line: Robeson upper bound (2008)17. Open squares: PIM-1 in literature; solid triangles: other PIMs in literature21,32,33,34,41, TZ-PIM20, PIM-SBF32, PIM-EA-TB21and PIM-SBI-TB21; open circles: TR polymers18,31,34,42,43,44; solid squares (black): unmodified PIM-1; solid squares (red): TOX-PIM-1 membranes. (h) CO2/CH4selectivity and (i) CO2/N2selectivity versus the fugacity of CO2for separation of gas mixtures (50/50 vol.%). The unmodified dense PIM-1 polymer membrane was annealed at 120 °C for 24 h under vacuum. The TOX-PIM-1 membrane in all panels was thermal-oxidatively crosslinked at 385 °C for 24 h under vacuum (1 mbar), the same condition as the sample shown inFig. 2c. Figure 3: Gas sorption and transport properties. ( a ) N 2 adsorption–desorption isotherms at 77 K. ( b ) Gas sorption isotherms at 273 K and ( c ) high-pressure gas sorption at 295 K (open symbols: PIM-1 membrane; solid symbols: TOX-PIM-1 membrane). ( d ) Permeability versus kinetic diameter of gases measured at 295 K. ( e ) Gas solubility (1 bar, 295 K) as a function of critical temperature ( T C ) of gas molecules. ( f ) Diffusivity as a function of square of effective molecular diameter ( d eff ) of gas molecules at 295 K. ( g ) Robeson plot of CO 2 /CH 4 selectivity versus CO 2 permeability. Commercial polymers are included for comparison: cellulose acetate (CA); ethyl cellulose (EC); polycarbonate (PC); Matrimid 5218 polyimide (PI); polyetherimide (PEI); polyphenyleneoxide (PPO); polysulphone (PSF), for comparison see ref. 40 . Upper bound line: Robeson upper bound (2008) [17] . Open squares: PIM-1 in literature; solid triangles: other PIMs in literature [21] , [32] , [33] , [34] , [41] , TZ-PIM [20] , PIM-SBF [32] , PIM-EA-TB [21] and PIM-SBI-TB [21] ; open circles: TR polymers [18] , [31] , [34] , [42] , [43] , [44] ; solid squares (black): unmodified PIM-1; solid squares (red): TOX-PIM-1 membranes. ( h ) CO 2 /CH 4 selectivity and ( i ) CO 2 /N 2 selectivity versus the fugacity of CO 2 for separation of gas mixtures (50/50 vol.%). The unmodified dense PIM-1 polymer membrane was annealed at 120 °C for 24 h under vacuum. The TOX-PIM-1 membrane in all panels was thermal-oxidatively crosslinked at 385 °C for 24 h under vacuum (1 mbar), the same condition as the sample shown in Fig. 2c . Full size image Gas transport properties Single-gas permeations through polymer membranes were performed at 295 K with industrially important gas molecules with different kinetic diameters, including H 2 (2.89 Å), CO 2 (3.3 Å), O 2 (3.46 Å), N 2 (3.64 Å) and CH 4 (3.8 Å), as shown in Fig. 3d . Gas transport in microporous PIM-1 polymer can still be illustrated with the solution diffusion model, where the permeability coefficient ( P ) is a product of solubility ( S ) and diffusion coefficient ( D ), P = S × D. The gas permeability of unmodified PIM-1 follows the sequence of CO 2 >H 2 >O 2 >CH 4 >N 2 , owing to the combined effects of sorption (for example, condensable CO 2 and CH 4 ) and diffusion (gas molecules with different sizes). After thermal-oxidative crosslinking at 385 °C under vacuum of 1 mbar, the TOX-PIM-1 membrane showed significantly lower gas permeability for larger molecules (N 2 and CH 4 ) by two orders of magnitude, while smaller gas molecules (H 2 , CO 2 , O 2 ) maintained considerably high permeability, giving a more remarkable molecular sieving function. Figure 3g shows a representative plot of selectivity versus permeability for an industrially important CO 2 /CH 4 gas pair along with the upper bound limit of polymer membranes. For a representative TOX-PIM-1 membrane crosslinked at 385 °C, the CO 2 /CH 4 selectivity increased up to 70 with a high CO 2 permeability of 1,100 Barrer (1 Barrer=1 × 10 −10 cm 3 cm cm −2 s −1 cm Hg −1 at standard temperature and pressure (STP)). The significantly enhanced gas selectivity along with high permeability push the overall gas transport properties to surpass the upper bound that has been limiting the polymer membranes for decades. To the best of our knowledge, the overall separation performance of TOX-PIM-1 membranes is higher than all existing soluble polymers including commercial polymers [40] , soluble PIMs [41] and compares very well against TR polymers [18] , [31] , [34] , [42] , [43] , [44] . The gas solubilities at 295 K and 1 bar are derived from the sorption isotherms ( Fig. 3c ) and correlate well with the critical temperature of gas molecules ( Fig. 3e ). Based on the solubility and gas permeability ( Fig. 3d ), gas diffusion coefficients (at 1 bar, 295 K) are derived as shown in Fig. 3f (detailed data are given in Supplementary Table 2 ), proving an evident shape-selective molecular sieving effect. The increase in diffusivity selectivity ( D A / D B ) and constant solubility selectivity ( S A / S B ) confirm that the significant improvement of gas selectivity is attributed to the structural modification of the gateways between the free volume cavities. The separation of gas mixtures was also examined for the TOX-PIM-1 membranes, including CO 2 /CH 4 and CO 2 /N 2 ( Supplementary Fig. 16 ). Figure 3h,i show the selectivity of CO 2 /CH 4 and CO 2 /N 2 versus CO 2 fugacity for separation of corresponding gas mixtures. In a mixed gas atmosphere, gas molecules compete for sorption sites, particularly at high pressure. Therefore, we observed a decrease in the CO 2 /CH 4 selectivity at high pressure, which nevertheless is still as high as 30 over CO 2 fugacity of 5–10 bar, a range of interest for industrial natural gas purification. In the case of CO 2 /N 2 separation, the selectivity is above 40 at low pressure of 2 bar while the CO 2 permeability is maintained above 1,000 Barrer. Such performance is of potential for efficient separation of CO 2 from flue gas emitted from coal-fired power plants at atmospheric pressure. Tunable gas transport properties We tuned the gas transport properties by controlling the degree of polymer crosslinking via controlling temperature ( Fig. 4a,b ), reaction time ( Fig. 4c,d ), and O 2 concentration ( Fig. 4e,f ). At excessive oxidative pyrolysis conditions (for example, weight loss about 3 wt% at 400 °C under vacuum), the CO 2 permeability shows a significant drop (<100 Barrer) and the gas transport properties became close to those of carbon molecular sieve membranes. In an extreme instance, by baking the polymer at 385 °C in air for 10 min (weight loss about 2.5 wt%), the CO 2 /CH 4 selectivity was also enhanced up to 70, while the CO 2 permeability maintained as high as ~500 Barrer, although the membrane became brittle due to excessive decay of mechanical properties. We summarize the gas transport properties obtained at various thermal oxidation conditions ( Supplementary Table 3 ). A typical Robeson plot of CO 2 /CH 4 selectivity versus CO 2 permeability in Fig. 4g shows the overall trends of significant enhancement of selectivity while the gas permeability decrease although maintaining at a significant level over commercial polymer membranes. 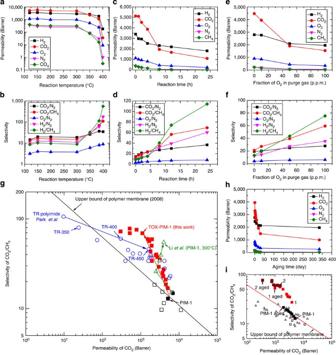Figure 4: Tunable gas transport properties. (a) Permeability and (b) selectivity as a function of annealing temperature under vacuum (1 mbar). All samples were thermally treated at set-point temperature for 24 h under vacuum, except that the sample at 400 °C was annealed for 12 h. (c) Permeability and (d) selectivity of PIM-1 membranes exposed to heat treatment at 385 °C under vacuum (1 mbar) for varied periods. (e) Permeability and (f) selectivity of membranes exposed to heat treatment at 385 °C in purging gas of argon containing p.p.m.-level O2. More data are given inSupplementary Table 3. (g) Robeson upper bound plot of CO2/CH4selectivity versus CO2permeability showing the trend of gas transport properties on exposure to thermal oxidative crosslinking. Arrows are added to guide the eyes. Data sets also include TR polymers by Parket al18, and thermally crosslinked PIM-1 membranes by Liet al.36(h) Change of gas transport properties of TOX-PIM-1 membranes under vacuum over 330 days. TOX-PIM-1 membrane was prepared by thermal-oxidative crosslinking at 385 °C in argon containing 10 p.p.m. O2. (i) Robeson plot showing the aging of PIM-1 (about 450 days) and TOX-PIM-1 membranes (about 330 days). Detailed data are given inSupplementary Fig. 17. Sample (1) and (2) correspond to membranes exposed to heat treatment at 385 °C for 24 h in argon containing 10 p.p.m. and 100 p.p.m. O2, respectively. Figure 4: Tunable gas transport properties. ( a ) Permeability and ( b ) selectivity as a function of annealing temperature under vacuum (1 mbar). All samples were thermally treated at set-point temperature for 24 h under vacuum, except that the sample at 400 °C was annealed for 12 h. ( c ) Permeability and ( d ) selectivity of PIM-1 membranes exposed to heat treatment at 385 °C under vacuum (1 mbar) for varied periods. ( e ) Permeability and ( f ) selectivity of membranes exposed to heat treatment at 385 °C in purging gas of argon containing p.p.m.-level O 2 . More data are given in Supplementary Table 3 . ( g ) Robeson upper bound plot of CO 2 /CH 4 selectivity versus CO 2 permeability showing the trend of gas transport properties on exposure to thermal oxidative crosslinking. Arrows are added to guide the eyes. Data sets also include TR polymers by Park et al [18] , and thermally crosslinked PIM-1 membranes by Li et al. [36] ( h ) Change of gas transport properties of TOX-PIM-1 membranes under vacuum over 330 days. TOX-PIM-1 membrane was prepared by thermal-oxidative crosslinking at 385 °C in argon containing 10 p.p.m. O 2 . ( i ) Robeson plot showing the aging of PIM-1 (about 450 days) and TOX-PIM-1 membranes (about 330 days). Detailed data are given in Supplementary Fig. 17 . Sample (1) and (2) correspond to membranes exposed to heat treatment at 385 °C for 24 h in argon containing 10 p.p.m. and 100 p.p.m. O 2 , respectively. Full size image The tunable gas transport properties of other industrially important gas pairs, such as O 2 /N 2 , CO 2 /N 2 , H 2 /N 2 and H 2 /CH 4 , follow similar trends as shown in Fig. 5 . For example, the O 2 /N 2 selectivity could be enhanced to as high as ~8.0 while the permeability remains as high as 250 Barrer. Such remarkable O 2 /N 2 separation performance is very promising for applications in N 2 separation or oxygen enrichment (for oxy-fuel combustion). The notable H 2 separation over N 2 and CH 4 are attractive for practical applications in H 2 recovery and natural gas purification. Interestingly, the gas transport data of TOX-PIM-1 membranes obtained from various experimental conditions seem to follow a continuous trend in the upper bound plot, in agreement with the tunable gas diffusivity and structural transformation of micropore structure. 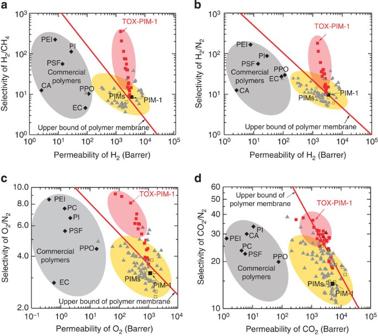Figure 5: Upper bound plot. Selectivity versus permeability of PIM-1 and TOX-PIM-1 membranes for industrially important gas pairs. (a) H2/CH4, (b) H2/N2(c) O2/N2and (d) CO2/N2. Red lines: State-of-the-art upper bound of polymer membrane summarized by Robeson in 2008 (ref.17). Commercial polymers (grey regions) are included for comparison. Open squares: PIM-1 in literature; solid triangles (yellow regions): other PIMs in literature21,32,33,34,41; solid squares (black): PIM-1 membrane; solid squares (red): representative TOX-PIM-1 membranes under different thermal oxidation conditions (detailed data are given inSupplementary Table 3). Figure 5: Upper bound plot. Selectivity versus permeability of PIM-1 and TOX-PIM-1 membranes for industrially important gas pairs. ( a ) H 2 /CH 4 , ( b ) H 2 /N 2 ( c ) O 2 /N 2 and ( d ) CO 2 /N 2 . Red lines: State-of-the-art upper bound of polymer membrane summarized by Robeson in 2008 (ref. 17 ). Commercial polymers (grey regions) are included for comparison. Open squares: PIM-1 in literature; solid triangles (yellow regions): other PIMs in literature [21] , [32] , [33] , [34] , [41] ; solid squares (black): PIM-1 membrane; solid squares (red): representative TOX-PIM-1 membranes under different thermal oxidation conditions (detailed data are given in Supplementary Table 3 ). Full size image Aging behaviour A particular concern for the use of glassy polymeric materials as gas separation membranes is their performance over several years, where the glassy polymer is expected to age. Thermodynamically, the rigid polymer chains still tend to pack space efficiently due to the relative freedom of conformation and rotation, and intermolecular non-covalent interactions (chain entanglements, hydrogen bonding, and so on) as the system tends to reach equilibrium. The gas permeability of PIM-1 shows gradual loss but at rates lower than other high free volume polymers, such as poly(1-trimethylsilyl-1-propyne) [45] , while the selectivity slightly increases under continuous vacuum. The aging of TOX-PIM-1 membranes followed a decrease in gas permeability and increase in selectivity under vacuum over initial 3–5 days, but then slowly stabilized over prolonged time of about 1 year ( Supplementary Fig. 17 ). Some representative data are shown for a representative CO 2 /CH 4 gas pair in Fig. 4h,i , confirming that the gas transport properties of aged crosslinked polymer network remained at a significant level. In a broader context, the crosslinked network may not suffer from chain conformational relaxation in other molecular level separations involving solvent swelling, such as pervaporation and organic solvent nanofiltration [46] . Thermal treatment of organic materials at high temperature involves complex chemical reactions (for example, pyrolysis, combustion, degradation, crosslinking, carbonization, and so on), heat and mass transfer and changes of physicochemical properties. Controlled thermal processing is widely used, such as pyrolysis, gasification and combustion of fuels, gasification and oxidation of biomass (or polymers and coal) in the presence of steam or O 2 for producing carbon molecular sieves (CMS) and activated carbon (dominant adsorbents). In the membrane field, Koros and co-workers [47] , [48] found the critical role of oxygen in controlling the atmosphere of pyrolysis to tailor the gas separation performance of CMS membranes (known as O 2 doping). However, the CMS membranes are normally heated at temperatures above 500 °C, consequently losing mechanical strength. Instead, thermochemical transformation at relatively lower temperature is desired to retain the mechanical strength. For example, a unique class of TR polymers were derived from polyimides (PIs) containing ortho-positioned functional groups (for example, -OH and -SH) by heating at 350–450 °C [18] . The TR polymers start from non-porous glassy PIs, through thermochemical reactions, to insoluble and infusible molecular sieving materials with hour-glass shaped micropore structure, while the gas transport properties change from the region of high selectivity/low permeability to significantly higher permeability and slight loss in selectivity ( Fig. 4g ). In contrast, our novel approach starts from microporous PIM-1 polymer precursor that is transformed to crosslinked polymer networks via thermal oxidative crosslinking reactions at intermediate temperatures, which are different from those reactions occurred in CMS (for example, controlled oxidation and carbonization at high temperature) or TR polymers (rearrangement). Our TOX-PIM-1 membranes showed remarkably enhanced selectivity while the gas permeability decreased but remained at a significant level that is two-to-three orders of magnitude higher than commercial polymers, for a number of gas pairs and comparable to that of CMS or TR membranes (see a summary of data in Supplementary Table 4 ). Sorption data shows little change in the overall solubility of gases, before and after thermal processing, indicating that mild chemical changes have taken place primarily at these gateways with minimal impact on the overall free volume. This is corroborated by the similar rates of aging, or chain conformation observed within the PIM-1 and the major portions of network TOX-PIM-1, albeit from different starting points on the Robeson plot ( Fig. 4i ). Therefore, the loss in permeability in the PIM-1 material and its enhanced selectivity arises from thermo-oxidative closure of the bottlenecks between high free volume domains. The novelty of our work on the controlled thermal oxidative crosslinking of the PIM-1 polymer is also different from the paper reported by Li et al. [36] on thermally treated PIM-1 polymer. The paper of Li et al. [36] describes a less well-controlled thermal processing of PIM-1 at temperature of 300 °C, and reported that both permeability and selectivity are enhanced (see Fig. 4g ) while inducing crosslinking without the generation of volatile side-products. In contrast, we find that membranes annealed at 300 °C under vacuum or inert atmosphere remain stable, with strong evidence from molecular weight distribution, IR spectra, TGA data and gas permeation data. In fact, the earliest work by Budd et al. [23] already found that PIM-1 is stable at temperature up to 450 °C in inert atmosphere (350 °C in air), even when heated at 300 °C for 24 h. It is also notable that Du et al. [49] were unable to reproduce the claims by Li et al. while using a higher temperature (375 °C) and shorter times (45 min). Du et al. indicated that the annealing time was not sufficiently long enough for crosslinking (likely owing to lower O 2 concentration in high purity inert purge gas), as proven by our kinetic study at 385 °C in Fig. 4c . According to the Arrhenius-like expression of oxidative degradation kinetics with temperature ( Supplementary Fig. 11 ), we believe it is highly unlikely that crosslinking reactions can occur at 300 °C within the two days that Li et al. have annealed their materials. Our extensive experimental data provide solid evidence supporting a different and more reasonable thermal oxidative degradation mechanism. Furthermore, our understandings of the phenomenon of thermal oxidative crosslinking of PIM-1 polymer allow us to precisely tune the reaction kinetics and the structure of micropores in the membrane, and consequently tailor the gas diffusivity and separation performance. The reaction mechanism merits more discussion. Recently, a decarboxylation-induced crosslinking mechanism has been proposed by Koros and co-workers [50] for carboxylic acid-containing PIs (at 389 °C in inert atmosphere), and carboxylated PIMs by Du et al and Guiver and co-workers [37] , [49] (at 375 °C in inert atmosphere). Both studies have proposed free radical-induced covalent crosslinking following the decarboxylation reactions. In this study, during thermal treatment at similar temperature range (over 350–400 °C, preferably 375–385 °C) in the presence of oxygen, oxidation and crosslinking occurred. It is generally acknowledged that thermal oxidation (and oxidation induced by light or ozone) of polymer involves free radical chain reactions, including initiation (for example, hydrogen abstraction or weak links along the chain), propagation and termination (for example, crosslinking) [51] . According to the well-known chain reaction mechanism [51] , the oxygen reacts with the free radical (R·) forming peroxy radical (ROO·), which can further abstract a hydrogen from adjacent polymer chain to generate hydroperoxide (ROOH). The unstable hydroperoxide can split into two free radicals (RO· and ·OH), which would continue to propagate to initiate new free radical chain reactions until termination occurs, such as crosslinking due to the combination of radical sites on adjacent chains. In the temperature window of 350–450 °C (or preferably, 350–400 °C), the possible reaction sites could involve the methyl groups, dioxane linkages and spiro-carbon centre, while the fused aromatic rings should be relatively more stable. The weaker methyl groups on the spiro-carbon centre are possible initial sites for abstraction of hydrogen. Mass balances obtained in TGA ( Fig. 2h ) confirmed that very little amount of weight loss (1.5–2.5 wt%) is sufficient to achieve high degree of crosslinking with excellent molecular sieving properties. The chemical formula for one repeating unit of PIM-1 is C 29 H 20 N 2 O 4 , corresponding a molecular weight of 460.5 g mol −1 . A little amount of weight loss up to 1.5–2.5 wt% corresponds to 7–11.5 g for 1 mol repeating unit, ideally, abstraction of several hydrogen atoms from the four methyl groups (-CH 3 , containing 12 H atoms), or abstraction of methyl radicals (·CH 3 ) would be sufficient. Of course, the evolution of molecular weight distribution indicates a mechanism of random scission involving the backbone, rather than simply abstraction of side groups. Therefore, mechanisms of both oxidative chain scission and covalent crosslinking merit further study in the future. In practice, polymer separation membranes can be fabricated using established techniques and module designs (flat sheet, spiral wound or hollow fibres) followed by post treatment. Indeed, many parameters are involved in the thermal oxidative crosslinking, including the temperature, oxygen concentration in the polymer and purge gas, heating rate and reaction time. But we demonstrate that these parameters could be carefully controlled in our experiments or more delicately controlled TGA-like reactor, using a chemical reaction engineering approach. We confirmed that the crosslinking through the thick PIM-1 polymer films could be achieved. We have also demonstrated that the oxidative crosslinking is effective for PIM-1 polymer thin films coated on silicon or glass substrates, which are dense and defect free as examined by SEM ( Supplementary Fig. 18 ). Similarly, we expect that thin films coated on thermally stable porous ceramic membrane supports can be exposed to heat treatment at controlled atmosphere, potentially allowing the scale up of our process. Because it is not possible to achieve a completely oxygen-free atmosphere in practice, trace amounts of oxygen absorbed in organic microporous materials can always induce oxidation on thermal processing and consequently resulting in significantly different properties. Our approach on PIM-1 polymer represents a rational design and transformation of PIMs polymers, which is of broader fundamental significance to post-synthetic modification of the structure of channels and pores in a wide range of porous materials, such as MOFs [52] , porous organic molecules [53] , [54] , [55] , [56] , covalent organic frameworks [57] and graphene-based carbon materials [58] , [59] , [60] . In summary, we report the phenomenon of thermo-oxidative degradation and crosslinking of PIM-1 polymer with a broad distribution of microporosity, and demonstrate rational control of this process to tune the micropore structure of membranes and molecular sieving functions. Our approach leads to highly permeable and selective membranes that show great potential for molecular level separations in energy and environmental processes, such as capturing CO 2 from flue gas, air separation, biogas and natural gas production, H 2 production, separation of hydrocarbons (olefin/paraffin) in petrochemical industries, pervaporation and organic solvent nanofiltration. In a broad context, our method is not limited to membrane applications, the controlled thermally crosslinked polymer frameworks can be used as molecular sieves for other applications, for example, solid sorbents for sorption of gas and chemicals. Furthermore, this broader principle is instructive in utilizing other porous polymeric materials and tuning the topology and structure of channels and pores for a wide range of applications. Synthesis of polymer The PIM-1 polymer was synthesized following the method invented by Budd et al. [23] , from polycondensation reaction of 3,3,3′,3′-tetramethyl-1,1′- spirobisindane-5,5′,6,6′-tetrol (TTSBI, 30 mmol, Alfa Aesar) and 2,3,5,6-tetrafluoroterephthalonitrile (TFTPN, 30 mmol, Matrix Scientific) in the presence of K 2 CO 3 (60 mmol, Aldrich) in anhydrous dimethylformamide (200 ml). After the mixture has been stirred at 60 °C for about 48 h, the polymer was purified by dissolving in chloroform and re-precipitation from methanol, filtered and dried in vacuum oven at 110 °C for overnight. The molecular weight of purified polymer was determined from gel permeation chromatography (GPC), giving an average molecular weight of M n =80,000 to 100,000 Da and a polydispersity of 2.0. Preparation of membranes Thick dense membranes were prepared by casting polymer solution in chloroform. Non-dissolved particles were removed by filtration through PTFE filters or by centrifugation. Polymer solutions were cast on clean glass substrate in a glove box. After the solvent has been slowly evaporated at room temperature in 2 days, the dry free-standing membranes were obtained and exposed to methanol soaking for overnight and dried in air. After, the membrane was dried in a vacuum oven at 120 °C for 24 h. Thin films were prepared by spin coating of diluted PIM-1 solution in chloroform on different substrates. Thermal analyses Thermal analyses of polymer films were performed in a TGA to study the thermal degradation and thermal oxidative degradation in well-controlled atmosphere. The gas species evolved from the TGA was analysed by a FTIR. The gas atmosphere includes Argon (Air products), Air (zero grade, air products) and O 2 /Argon mixture (200 p.p.m. O 2 , balance argon, BOC). In one series of experiments, polymer films were dynamically heated from room temperature to 1,000 °C at 10 °C min −1 in inert atmosphere or in air. Another series of experiments were carried out using O 2 /Argon mixture (200 p.p.m. O 2 , balance argon, BOC). A batch of dense polymer films (~5 mg, dimension of 3 × 3 mm) were heated at 120 °C for 1 h under continuous flow of purging gas to remove moisture and residual gases, then heated at 10 °C min −1 to varied temperature (300–450 °C), then kept at the set-point temperature for 2 h. Thermal oxidative crosslinking The PIM-1 membranes were exposed to thermal treatment under controlled atmosphere in a high temperature vacuum oven (Heraeus, 20–400 °C). The vacuum oven was modified allowing operation in controlled vacuum or purging mode. The pressure was monitored continuously by pressure transmitters (Keller, UK). A series of experiments were performed by heating the polymer at different temperature under continuous controlled vacuum (1 mbar). Flat polymer films were placed on the plate in the vacuum oven and heated under vacuum at 120 °C for 3 h, then heated to final temperature at 10 °C min −1 . Then the samples were maintained at the temperature for extended time up to 24 h. Another series of experiments were carried out by heating PIM-1 membranes in the vacuum oven at 385 °C, with the vacuum pressure controlled at 1, 10, 20, 50, 100, 200 mbar. Alternatively, we controlled the atmosphere of heat treatment by purging inert gases containing low concentrations of O 2 (0–200 p.p.m. ), including high purity argon (B.I.P. grade, O 2 <10 p.p.b., air products) and O 2 balanced with argon (BOC, UK), with nominal O 2 concentration at 10 (9.2), 50 (55), 100 (104), 200 (215) p.p.m., where the value in parentheses are the calibrated concentration. The flow rate (2 l min −1 ) was controlled by a metering valve. The polymer films were placed on the heating plate in the oven, and exposed to vacuum at 120 °C under vacuum for 1 h, then purging gas was introduced to the oven to pressurize the oven close to 1,000 mbar, then vacuum was switched on again to reduce the pressure. After at least five cycles of vacuum pressurization, the samples were exposed to continuous flow of purging gas for a certain period. In extreme cases, the polymer films were simply baked in air. In one series of experiment, the polymer films were heated in air from 120 °C to 385 °C at 10 °C min −1 . Rapid change of colour from fluorescent yellow to brownish was observed when the temperature was above 350 °C. During this heating stage, the polymer films were turned over frequently, manually with tweezers. When the temperature reached to 385 °C, the brown colour thermally oxidized polymer films were removed from the oven to avoid excessive degree of degradation (too brittle for gas permeation tests) due to the fast reaction rate as shown in TGA (as evidenced by further colour changing to black) and cooled down naturally to ambient temperature. Alternatively, the oven was switched to vacuum mode. In the mean time, the power of the oven was turned off allowing the films to cool down to room temperature under vacuum. In another series of isothermal experiment, fresh membranes were moved from ambient condition to the preheated oven (385 °C) and baked for 10 min, and removed from the oven immediately. The three methods gave similar degrees of degradation of polymer, with weight loss at ~2.5 wt%. The volatile products released should be connected to ventilation. Characterization SEM analysis of membranes was performed using a Hitachi S5500 microscope. The polymer films were fractured in liquid nitrogen and coated with a thin layer of gold. The molecular weight of polymer was quantified by GPC calibrated with polystyrene standards. Ultraviolet–visible absorption spectra of polymer thin film (~100 nm,) were measured using a Hewlett Packard 8453 Ultraviolet–visible spectrometer. Steady-state photoluminescence excitation measurements were measured with a CARY Eclipse fluorescence spectrophotometer, at an excitation wavelength of 420 nm. The FTIR spectra were measured using an infrared spectrometer in transmission mode, or using an attenuated total reflectance cell. The skeletal density of polymer films (100–200 mg) was measured using a Micromeritics Accupyc 1340 helium pycnometer. Before density measurements, all samples were evacuated thoroughly under vacuum at 150 °C for 5 h. The apparent bulk density was measured from the gravimetric method, using films with uniform thickness and quantifying the mass and size. The gel fractions of crosslinked polymer films were quantified by soaking them in solvent and the weight fraction of undissolved gel was quantified, while the dissolved fraction of polymer was examined with GPC to quantify the evolution of molecular weight distribution. Wide-angle X-ray scattering was performed with a Bruker D8 machine operated at 40 mA and 40 kV using Cu Kα radiation with a step of 0.02° per second. Mechanical properties Tensile tests of polymer films were carried out at a home-made stretcher machine. Polymer films with thickness in the range of 50–80 μm were cut into thin slices with an effective length of ~20 mm and a width of ~2 mm, with the accurate value determined from high-resolution photos and calibrations from known length. The films were stretched for 0.02 mm in each step with a relaxation time of 30 s, giving an apparent strain rate of ~4 × 10 −5 s −1 . The average value of Young’s modulus was derived from the initial slope. The tensile strength at break and elongation at break were also measured. Nanoindentation of surfaces of polymer membranes were performed at ambient temperature using a sharp Berkovich tip in the continuous stiffness measurement mode on an MTS NanoIndenter XP (MTS, Eden Prairie, MN). The indenter axes were aligned normal to the membrane planes. The average values of the Young’s modulus ( E ) and the hardness ( H ) were extracted from the force–displacement P–h curves over depths of 100–1,000 nm, with a series of 20 measurements at different locations. Gas sorption Low-pressure gas sorption was performed using a Micromeritics ASAP 2020 instrument at pressures up to 1 bar. Dense polymer membranes (~0.1 g) with thickness of ~50 μm were cut into small pieces, loaded into the apparatus and degassed at 120 °C under high vacuum(<10 −6 bar). After the mass had been measured, the samples were further degassed under high vacuum for the gas sorption measurement. Nitrogen adsorption–desorption isotherms were measured at 77 K and 273 K, respectively. The sorption isotherms of CO 2 and CH 4 were also measured at 273 K. The specific surface area was calculated based on the Brunauer-Emmett-Teller model and the pore size distribution was derived from non-local density functional theory model from N 2 isotherms at 77 K or from CO 2 sorption isotherms at 273 K when the sorption of N 2 was subjected to kinetic control. High-pressure pure-gas sorption isotherms were measured using a home-made dual-volume pressure decay apparatus at pressures up to 35 bar and at 295 K. A batch of polymer films was heated at 120 °C under high vacuum for 12 h. After measurement of the mass, the films were loaded in the sample cell and further evacuated for 12 h before sorption measurements. The amount of gas sorption was calculated from the mass balance of gas molecules based on the equation of gas states, using the equilibrium pressure calibrated with compressibility factors. The measurements followed the sequence of H 2 , O 2 , N 2 , CH 4 and CO 2 . The samples were thoroughly evacuated between measurements of each gas. Gas permeation Pure gas permeation tests were carried out at temperature of 22 °C and feed pressure of 4 bar, using a constant-volume pressure-increase apparatus. The mixed gas permeation properties were measured in another membrane cell using the constant-pressure variable-volume method. The membrane was exposed to certified gas mixtures (BOC, UK) of CO 2 /CH 4 (50/50 vol.%) and CO 2 /N 2 (50/50 vol.%) with feed pressures up to 35 bar at room temperature (22 °C), with a stage cut (ratio of flow rates of permeate to feed) less than 1%. The gas compositions were analysed by a gas chromatograph (GC-2014, Shimadzu). Details are given in the Supplementary Methods . Molecular simulation Molecular dynamics (MD) simulations were performed with the Materials Studio software package (Accelrys, CA, USA). In one amorphous cell, four PIM-1 polymer chains with 10 repeating units were constructed at 298 K. For the thermally oxidized and crosslinked polymers, the reaction mechanisms are very complicated. Here, we use the MD simulation primarily to understand the intermolecular interactions (for example, hydrogen bonding), and packing of short polymer segments. To mimic the oxidative chain scission, 20 short chains containing two repeating units of PIM-1 with oxidized groups (for example, carboxylic acid groups, -COOH) were constructed in another amorphous cell at 298 K as well. Covalently crosslinked polymers were not simulated, due to the difficulty to analyse the chemical structure. The Berendsen algorithm with a decay constant of 0.1 ps was used to control the temperature and pressure of each cell. The specific procedures are as follows: (1) energy minimization; (2) 50 ps NVT-MD simulation at 600 K; (3) 50 ps NPT-MD simulation at 600 K at 1 bar; (4) 50 ps NPT-MD simulation at 298 K at 1 bar; (5) 50 ps NPT-MD simulation at 298 K at 10 bar with a step of 1.0 fs; (6) 50 ps NVT-MD at 298 K; (7) 50 ps NPT at 298 K at 1 bar. The Ewald summation method was used to calculate the non-bond interactions with an accuracy of 0.001 kcal mol −1 . Hydrogen bonding was automatically monitored by the software based on a list of hydrogen-bonding scheme (N, O, S, and halogens). How to cite this article: Song, Q. et al. Controlled thermal oxidative crosslinking of polymers of intrinsic microporosity towards tunable molecular sieve membranes. Nat. Commun. 5:4813 doi: 10.1038/ncomms5813 (2014).